Pre-anaphase chromosome oscillations are regulated by the antagonistic activities of Cdk1 and PP1 on Kif18A Upon congression at the spindle equator, vertebrate chromosomes display oscillatory movements which typically decline as cells progress towards anaphase. Kinesin-8 Kif18A has been identified as a suppressor of chromosome movements, but how its activity is temporally regulated to dampen chromosome oscillations before anaphase onset remained mysterious. Here, we identify a regulatory network composed of cyclin-dependent kinase-1 (Cdk1) and protein phosphatase-1 (PP1) that antagonistically regulate Kif18A. Cdk1-mediated inhibitory phosphorylation of Kif18A promotes chromosome oscillations in early metaphase. PP1 induces metaphase plate thinning by directly dephosphorylating Kif18A. Chromosome attachment induces Cdk1 inactivation and kinetochore recruitment of PP1α/γ. Thus, we propose that chromosome biorientation mediates the alignment of chromosomes at the metaphase plate by tipping the balance in favour of dephosphorylated Kif18A capable of suppressing the oscillatory movements of chromosomes. Notably, interfering with chromosome oscillations severely impairs the fidelity of sister chromatid segregation demonstrating the importance of timely controlled chromosome dynamics for the maintenance of genome integrity. During the different phases of mitosis, chromosomes undergo a series of well-defined movements. Upon nuclear envelope breakdown (NEBD), chromosomes attach to the forming spindle and move towards the spindle equator [1] . This motion termed congression [2] results in the alignment of chromosomes at the metaphase plate midway between the two spindle poles. In mammalian cells, bioriented chromosomes do not rest at the spindle equator but display oscillatory movements along the spindle axis. These oscillatory movements are confined to a narrow region around the spindle equator and characterized by their rough constant speed and abrupt directional switches [3] , [3] . As suggested previously [5] , changes in directional movement could enable chromosomes to evade obstacles within the densely packed mitotic spindle and, thereby, protect them from becoming damaged or entangled. However, as cells progress towards anaphase chromosome oscillations have to decline to mediate metaphase plate thinning resulting in the tight positioning of chromosomes at the spindle equator [4] , [6] . Upon dissociation of chromosome cohesion, sister chromatids are pulled towards opposite poles and partitioned into the two nascent daughter cells. The oscillatory movements of bioriented chromosomes are coupled to the coordinated dynamics of microtubules (MTs) attached to the two sister kinetochores (KTs). MTs attached to the leading KT have to depolymerize while MTs attached to the trailing KT must be in a polymerization state [7] , [8] . Kinesin-8 motors are characterized by their ability to affect MT dynamics [9] , [10] , [11] making them attractive candidates to control chromosome movements. Indeed, human Kinesin-8 Kif18A has been shown to limit the oscillation amplitude of chromosomes by decreasing their oscillation speed [4] , [12] . According to the current model, Kif18A due to its exceptional high processivity and long dwell time at MT plus-ends, which both depend on an additional MT binding site in the C-terminus of Kif18A [12] , [13] , [14] , [15] , accumulates at the tips of KT-MTs where it suppresses their dynamics and, thereby, limits the oscillation amplitude of chromosomes [10] , [16] . However, the question of how Kif18A activity is regulated to timely induce plate thinning remained elusive. Here, we show that chromosome oscillations are regulated by the inhibitory effect of cyclin-dependent kinase-1 (Cdk1) on Kif18A and the antagonistic activity of protein phosphatase-1 (PP1)α/γ. Reportedly, correct chromosome attachment has opposing effects on Cdk1 and PP1 function: It triggers Cdk1 inactivation by silencing the spindle assembly checkpoint (SAC) resulting in anaphase-promoting complex/cyclosome (APC/C) mediated destruction of cyclin B [17] and, at the same time, induces KNL1-mediated recruitment of PP1α/γ to outer KTs [18] . Altering chromosome oscillations by expressing Kif18A variants not responsive to Cdk1 and/or PP1 regulation severely impairs the fidelity of chromosome segregation. Therefore, based on our discoveries, we propose a model according to which chromosome biorientation promotes faithful sister chromatid segregation by inducing Kif18A-mediated suppression of chromosome oscillations resulting in the tight alignment of chromosomes at the metaphase plate. Cdk1 phosphorylates Kif18A at serine-674 and serine-684 To investigate the process of metaphase plate thinning, we analysed by time-lapse microscopy HeLa cells stably expressing CENP-A fused to mCherry and inducibly expressing green fluorescent protein (GFP)-tagged cyclin B1. As shown previously [19] , GFP-cyclin B1 levels started to decline upon alignment of all chromosomes at the metaphase plate ( Fig. 1a and Supplementary Movie 1 ). Notably, the decline in GFP-cyclin B1 coincided with metaphase plate thinning ( Fig. 1b and Supplementary Fig. 1a ) suggesting that Cdk1 inactivation might be critical for reduced chromosome oscillations in pre-anaphase cells. Since Kif18A limits the oscillatory movements of chromosomes [4] , [12] , we further speculated that Cdk1 controls the chromosome movements by regulating Kif18A. To test this hypothesis, we investigated if Kif18A is a Cdk1 substrate. SDS-polyacrylamide gel electrophoresis analyses revealed that Kif18A is phosphorylated in mitosis as evident by the appearance of a slower migrating form of Kif18A which upon treatment of cell extract with calf intestinal phosphatase (CIP) was converted into the faster migrating form ( Fig. 1c ). Notably, treatment of mitotic cells with roscovitine also resulted in the enrichment of the faster migrating form ( Fig. 1c ) suggesting that Kif18A is phosphorylated by Cdk1. To test if Cdk1/cyclin B rather than Cdk1/cyclin A is the roscovitine-sensitive kinase that phosphorylates Kif18A, we analysed the electrophoretic mobility of Kif18A derived from mitotic cells depleted of cyclin A2, the main A-type cyclin present in somatic cells [20] . Thymidine presynchronized cells were treated for 16 h with nocodazole and collected by shake-off. Consistent with previous reports [21] , Cdc27 immunoblot confirmed that cells depleted of cyclin A2 were able to enter mitosis ( Fig. 1d ). Importantly, depletion of cyclin A2 did not significantly affect the appearance of the slower migrating form of Kif18A ( Fig. 1d ) suggesting that Cdk1/cyclin B is the kinase that phosphorylates Kif18A in mitosis. To test if Kif18A is a direct Cdk1/cyclin B1 substrate, in vitro kinase assays using glutathione-S-transferase (GST) tagged N-terminal (NT, amino acid (aa) 1–592) and C-terminal (CT, aa 593–898) fragments of Kif18A were performed. Autoradiogram analysis revealed that Cdk1/cyclin B1 efficiently phosphorylated the C-terminus but not N-terminus of GST-Kif18A ( Fig. 1e ). Mass spectrometric analysis of in vitro phosphorylated GST-Kif18A CT identified serine (S) residues 674 and 684 as Cdk1 phosphorylation sites ( Fig. 1f ). Consistent with previous phospho-proteome analysis [22] , we exclusively identified peptides where both serine residues were phosphorylated. Autoradiogram analysis of in vitro kinase assays using wildtype (WT) and non-phosphorylatable (S674A/S684A→2A) GST-Kif18A CT verified these two serine residues as major Cdk1/cyclin B1 phosphorylation sites ( Fig. 1g ). 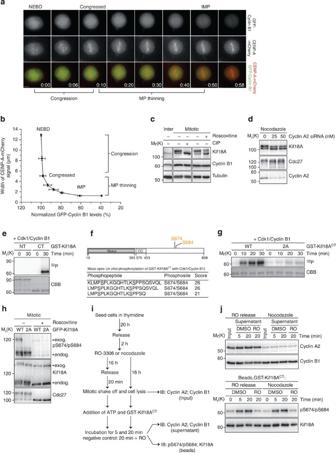Figure 1: Kif18A is a Cdk1 substrate. (a) Time-lapse images of HeLa cells stably expressing CENP-A-mCherry (red) and inducibly expressing GFP-cyclin B1 (green) used for quantifications shown inb. Time stamp at NEBD was set to 0:00 minutes. Time points for chromosome congression (Congressed) and tMP are depicted. Scale bar, 5.6 μm. See alsoSupplementary Movie 1. (b) Correlation of metaphase plate width—represented by CENP-A-mCherry signal—with GFP-cyclin B1 levels. GFP-cyclin B1 levels were normalized to 100% at NEBD. Mean±s.d. from two independent experiments withn=233 cells are shown. See alsoSupplementary Fig. 1a. (c) Interphase and mitotic (nocodazole release into MG132) cells were immunoblotted for Kif18A, cyclin B1 (mitotic marker) and tubulin (loading control). Cells were treated with roscovitine and cell lysate with CIP. (d) Cyclin A2-depleted cells were arrested in nocodazole and immunoblotted for Kif18A, Cdc27 and cyclin A2. (e)In vitroCdk1/cyclin B1 kinase assay using GST-Kif18A fragments 1–592 (NT) and 593–898 (CT) as substrate. Autoradiogram showing incorporation of γ-32P and coomassie staining (CBB) of purified proteins. (f) Schematic representation of the domain architecture of Kif18A and summary of the mass spectrometry analysis ofin vitroCdk1/cyclin B1 phosphorylated GST-Kif18ACT. Highlighted in orange are the two relevant phosphorylation sites S674 and S684. (g)In vitroCdk1/cyclin B1 kinase assay using WT or non-phosphorylatable (2A, S674A/S684A) GST-Kif18ACTas substrate. Autoradiogram showing incorporation of γ-32P and CBB of purified proteins. (h) Cells inducibly expressing GFP-Kif18AWTor GFP-Kif18A2Awere treated as incand immunoblotted for phosphorylated Kif18A (pS674/pS684), Kif18A and Cdc27. Cdk1 substrate Cdc27 serves as control for roscovitine treatment. See alsoSupplementary Fig. 1b. (i) Experimental outline ofin vitrokinase assay with GST-Kif18ACTas substrate incubated with cell extract containing different cyclin A2 levels. (j) GST-Kif18ACTwas incubated with cell extract containing high (RO-release) or low (nocodazole) cyclin A2 levels for the indicated time points and immunoblotted for pS674/pS684 and Kif18A. Input and supernatant samples were blotted for cyclin A2 and cyclin B1. Immunoblots showing the specificity of the pS674 and pS684 Kif18A antibodies are shown inSupplementary Fig. 1c. Figure 1: Kif18A is a Cdk1 substrate. ( a ) Time-lapse images of HeLa cells stably expressing CENP-A-mCherry (red) and inducibly expressing GFP-cyclin B1 (green) used for quantifications shown in b . Time stamp at NEBD was set to 0:00 minutes. Time points for chromosome congression (Congressed) and tMP are depicted. Scale bar, 5.6 μm. See also Supplementary Movie 1 . ( b ) Correlation of metaphase plate width—represented by CENP-A-mCherry signal—with GFP-cyclin B1 levels. GFP-cyclin B1 levels were normalized to 100% at NEBD. Mean±s.d. from two independent experiments with n =233 cells are shown. See also Supplementary Fig. 1a . ( c ) Interphase and mitotic (nocodazole release into MG132) cells were immunoblotted for Kif18A, cyclin B1 (mitotic marker) and tubulin (loading control). Cells were treated with roscovitine and cell lysate with CIP. ( d ) Cyclin A2-depleted cells were arrested in nocodazole and immunoblotted for Kif18A, Cdc27 and cyclin A2. ( e ) In vitro Cdk1/cyclin B1 kinase assay using GST-Kif18A fragments 1–592 (NT) and 593–898 (CT) as substrate. Autoradiogram showing incorporation of γ- 32 P and coomassie staining (CBB) of purified proteins. ( f ) Schematic representation of the domain architecture of Kif18A and summary of the mass spectrometry analysis of in vitro Cdk1/cyclin B1 phosphorylated GST-Kif18A CT . Highlighted in orange are the two relevant phosphorylation sites S674 and S684. ( g ) In vitro Cdk1/cyclin B1 kinase assay using WT or non-phosphorylatable (2A, S674A/S684A) GST-Kif18A CT as substrate. Autoradiogram showing incorporation of γ- 32 P and CBB of purified proteins. ( h ) Cells inducibly expressing GFP-Kif18A WT or GFP-Kif18A 2A were treated as in c and immunoblotted for phosphorylated Kif18A (pS674/pS684), Kif18A and Cdc27. Cdk1 substrate Cdc27 serves as control for roscovitine treatment. See also Supplementary Fig. 1b . ( i ) Experimental outline of in vitro kinase assay with GST-Kif18A CT as substrate incubated with cell extract containing different cyclin A2 levels. ( j ) GST-Kif18A CT was incubated with cell extract containing high (RO-release) or low (nocodazole) cyclin A2 levels for the indicated time points and immunoblotted for pS674/pS684 and Kif18A. Input and supernatant samples were blotted for cyclin A2 and cyclin B1. Immunoblots showing the specificity of the pS674 and pS684 Kif18A antibodies are shown in Supplementary Fig. 1c . Full size image To analyse if Cdk1 phosphorylates these sites in cells, we generated phospho-specific pS674 and pS684 antibodies. Immunoblot analyses of a ‘tetracycline-on’ HeLa cell line that on induction, stably expressed siRNA-resistant GFP-Kif18A (HeLa-Flp-In/T-REx) confirmed the specificity of the antibodies for pS674 and pS684 because the depletion of endogenous Kif18A resulted in the loss of the pS674/pS684 signal, GFP-tagged Kif18A WT but not Kif18A 2A was detected upon induction in mitotic cells, and the signal for endogenous as well as GFP-Kif18A WT disappeared upon lambda phosphatase treatment of mitotic cell lysate ( Supplementary Fig. 1b ). Consequently, incubation of Cdk1/cyclin B1 with WT but not 2A GST-Kif18A CT resulted in pS674/pS684 reactive signals ( Supplementary Fig. 1c ). Importantly, treatment of cells with roscovitine resulted in the loss of pS674/pS684 signal for both endogenous Kif18A and GFP-Kif18A WT ( Fig. 1h ). To further confirm the finding that Cdk1/cyclin B1 is the relevant kinase, recombinant GST-Kif18A CT was incubated in cell extracts containing high or low cyclin A2 levels and immunoblotted for pS674/pS684 ( Fig. 1i ). Early mitotic extract obtained by shake-off of cells released for 20 min from a RO-3306 induced G2-arrest [23] , contained high levels of both cyclin A2 and cyclin B1 ( Fig. 1j ). As expected, cyclin A2 was barely detectable in cells arrested in prometaphase for 16 h by nocodazole treatment, whereas cyclin B1 levels remained high ( Fig.1j ). Importantly, S674/S684 phosphorylation of GST-Kif18A CT was equally efficient in both extracts. Thus, while we cannot formally exclude the possibility that Cdk1/cyclin A2 might contribute to Kif18A phosphorylation in early mitosis, our experimental data indicate that Cdk1 in complex with cyclin B1 is the relevant kinase that phosphorylates Kif18A at S674/S684. Kif18A 2A induces metaphase plate thinning prematurely To test whether Cdk1 phosphorylation of Kif18A affects chromosome oscillations, we monitored chromosome movements in cells stably expressing CENP-A-mCherry together with WT or non-phosphorylatable 2A GFP-Kif18A. Unless otherwise stated, these studies like all further functional analyses were performed in the Kif18A depletion background using the aforementioned Flp-In/T-REx HeLa cell line. Following the outlined protocol ( Fig. 2a ), Kif18A was efficiently depleted ( Fig. 2b ) which as reported previously [24] caused a strong mitotic delay in cells not expressing GFP-Kif18A ( Supplementary Fig. 1d ). Upon induction, GFP-Kif18A WT and -Kif18A 2A were expressed at physiological levels ( Fig. 2b ). Using NEBD as the reference point, time-lapse analyses revealed that both WT- and 2A-expressing Kif18A-RNAi cells displayed similar timing for chromosome congression ( t CON : 7.1±1.1 min and 7.3±1.4 min (mean±s.d. ); Fig. 2c,d and Supplementary Movie 2 ). Intriguingly, however, once chromosomes have congressed to the metaphase plate, GFP-Kif18A 2A -expressing cells established a thin metaphase plate (tMP) significantly earlier than WT-expressing cells: (19.5±3.3 min versus 10.2±2.4 min; P =0.02; Fig. 2c,d and Supplementary Movie 2 ). Importantly, the final width of the thinnest metaphase plate was identical in WT- and 2A-expressing Kif18A-RNAi cells and remained constant until anaphase onset ( Fig. 2e ). WT-expressing cells entered anaphase about 34.6 min±2.5 min after NEBD, whereas 2A-expressing cells showed a subtle delay of about 10 min (44.4±6.0 min; Fig. 2d ). Depletion of Mad2 completely abolished this delay ( Supplementary Fig. 1f ) indicating that expression of GFP-Kif18A 2A interferes with timely SAC inactivation. 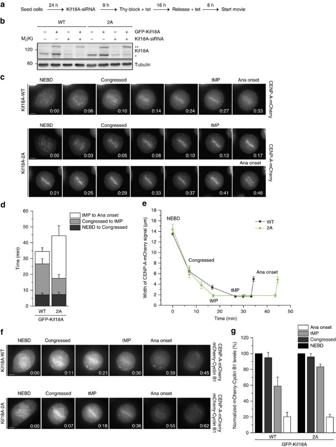Figure 2: Non-phosphorylatable GFP-Kif18A2Aaccelerates tMP formation. (a) Experimental outline of the Kif18A-RNAi rescue experiments. (b) Immunoblot showing the depletion of endogenous Kif18A by siRNA and tetracycline-induced, stable expression of GFP-Kif18A variants. One and two asterisks mark endogenous Kif18A and GFP-Kif18A, respectively. (c) Still images of movies showing KT movements marked by CENP-A-mCherry in Kif18A-RNAi cells inducibly expressing GFP-Kif18AWTand GFP-Kif18A2A. Time stamp at NEBD was set to 0:00 minutes. Scale bar, 5.6 μm. See alsoSupplementary Movie 2. (d) Quantification ofcusing three categories: Time from NEBD to chromosome alignment at the spindle equator (Congressed), from congression to establishment of a tMP and from formation of a tMP to anaphase onset (Ana onset). Bars represent the mean of three independent experiments withn=111 cells for WT andn=116 cells for 2A. Error bars represent s.d. See alsoSupplementary Fig. 1d,e. (e) Quantification ofcillustrating changes in the width of the metaphase plate—determined by CENP-A-mCherry signal—over time. Mean±s.d. are shown. (f) Time-lapse images showing HeLa cells inducibly expressing WT or 2A GFP-Kif18A and CENP-A-mCherry transiently transfected with mCherry-cyclin B1. Time stamp at NEBD was set to 0:00 minutes. Scale bar, 5.6 μm. See alsoSupplementary Movie 3. (g) Quantification of mCherry-cyclin B1 levels at indicated mitotic stages from cells shown inf. mCherry-cyclin B1 levels at NEBD were set to 100%. Bars represent the mean±s.d. from three independent experiments withn=25 cells for WT andn=26 cells for 2A. Figure 2: Non-phosphorylatable GFP-Kif18A 2A accelerates tMP formation. ( a ) Experimental outline of the Kif18A-RNAi rescue experiments. ( b ) Immunoblot showing the depletion of endogenous Kif18A by siRNA and tetracycline-induced, stable expression of GFP-Kif18A variants. One and two asterisks mark endogenous Kif18A and GFP-Kif18A, respectively. ( c ) Still images of movies showing KT movements marked by CENP-A-mCherry in Kif18A-RNAi cells inducibly expressing GFP-Kif18A WT and GFP-Kif18A 2A . Time stamp at NEBD was set to 0:00 minutes. Scale bar, 5.6 μm. See also Supplementary Movie 2 . ( d ) Quantification of c using three categories: Time from NEBD to chromosome alignment at the spindle equator (Congressed), from congression to establishment of a tMP and from formation of a tMP to anaphase onset (Ana onset). Bars represent the mean of three independent experiments with n =111 cells for WT and n =116 cells for 2A. Error bars represent s.d. See also Supplementary Fig. 1d,e . ( e ) Quantification of c illustrating changes in the width of the metaphase plate—determined by CENP-A-mCherry signal—over time. Mean±s.d. are shown. ( f ) Time-lapse images showing HeLa cells inducibly expressing WT or 2A GFP-Kif18A and CENP-A-mCherry transiently transfected with mCherry-cyclin B1. Time stamp at NEBD was set to 0:00 minutes. Scale bar, 5.6 μm. See also Supplementary Movie 3 . ( g ) Quantification of mCherry-cyclin B1 levels at indicated mitotic stages from cells shown in f . mCherry-cyclin B1 levels at NEBD were set to 100%. Bars represent the mean±s.d. from three independent experiments with n =25 cells for WT and n =26 cells for 2A. Full size image The overexpression of Kif18A reduces chromosome oscillations [12] implicating that differences in the expression levels of WT and 2A Kif18A could potentially contribute to the observed plate thinning phenotype. However, based on the following data, we can exclude this possibility: First, both WT and 2A Kif18A were expressed at physiological and, importantly, comparable levels in Kif18A-RNAi cells ( Fig. 2b ). Second, expression of GFP-Kif18A WT in cells not depleted of endogenous Kif18A did not affect timing of metaphase plate thinning ( Supplementary Fig. 1d ) demonstrating that Kif18A cannot be expressed to such high levels in our stable cell lines to induce overexpression artefacts. Together, these data indicate that the ability of GFP-Kif18A 2A to establish a tMP earlier in mitosis is due to intrinsic properties of non-phosphorylatable Kif18A. Indeed, when we correlated plate thinning with cyclin B1 levels, we observed that expression of GFP-Kif18A 2A enabled Kif18A-RNAi cells to establish a tMP at significantly higher mCherry-cyclin B1 levels than WT-expressing cells ( Fig. 2f,g and Supplementary Movie 3 ). Collectively, these data indicate that Cdk1 phosphorylation of S674/S684 negatively affects metaphase plate thinning. Protein phosphatase-1 dephosphorylates Kif18A at S674/S684 Metaphase plate thinning occurs as cells progress towards anaphase implicating the existence of a phosphatase that counteracts Cdk1 phosphorylation of Kif18A. Previous studies revealed that Klp5/Klp6, the fission yeast Kinesin-8, contain a conserved motif (R/KxVxF/W; x denoting any aa) that mediates binding to protein phosphatase-1 (PP1) [25] . To test the idea that PP1 is the phosphatase that antagonizes Cdk1, we first analysed if Kif18A interacts with PP1. Indeed, endogenous Kif18A co-purified with GFP-PP1α and GFP-PP1γ immunoprecipitated from mitotic cells but not with the GFP control ( Fig. 3a and Supplementary Fig. 1g ). In vitro pull-down experiments revealed that the interaction was direct and dependent on the PP1-binding motif as recombinant full-length His-PP1α and -PP1γ efficiently bound to GST-Kif18A CT,WT but not to GST-Kif18A CT mutated in the PP1-binding motif (KVVVW 616 →KVAVA 616 , PP1Δ; Fig. 3b,c ). As expected, non-phosphorylatable GST-Kif18A CT,2A efficiently associated with His-PP1α and -PP1γ, while the double mutant (PP1Δ+2A) failed to interact ( Fig. 3b,c ). Next, we analysed if PP1α and PP1γ can directly dephosphorylate Kif18A ( Fig. 3d ). Indeed, incubation of GST-Kif18A CT,WT prephosphorylated by Cdk1/cyclin B1 with His-PP1α or -PP1γ resulted in a significant reduction of the pS674/pS684 signal compared to the buffer control ( Fig. 3e ). Importantly, His-PP1α and -PP1γ failed to dephosphorylate GST-Kif18A CT,PP1Δ that was deficient in PP1-binding ( Fig. 3f ). In summary, these results demonstrate that PP1α and PP1γ dephosphorylate Kif18A at S674/S684 in a reaction that depends on a conserved PP1-binding motif located in the C-terminus of Kif18A. 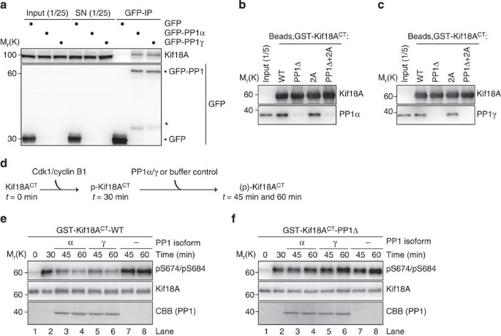Figure 3: PP1α and PP1γ dephosphorylate Kif18A at S674 and S684. (a) GFP and Kif18A immunoblots of input samples, supernatant (SN), and GFP immunoprecipitates (IP) from mitotic (nocodazole release in MG132) cells transfected with GFP, GFP-PP1α or GFP-PP1γ. Asterisk indicates unspecific band. A long exposure of the GFP immunoblot is shown inSupplementary Fig. 1g. (b) and (c)In vitropull-down assays using WT, PP1-binding deficient (PP1Δ), non-phosphorylatable (2A), and double defective (PP1Δ+2A) GST-Kif18ACT. Kif18A and PP1 immunoblots showing input and bead bound GST-Kif18ACTassociated with His-PP1α (b) or His-PP1γ (c). (d) Experimental outline ofin vitroPP1 phosphatase assays: GST-Kif18ACTwas prephosphorylated by incubation with Cdk1/cyclin B1 and the PP1 isoforms or buffer control were added to the kinase reaction without removing Cdk1/cyclin B1. (e) and (f)In vitroCdk1/cyclin B1 phosphorylated WT (e) and PP1 binding deficient (PP1Δ) (f) GST-Kif18ACTwere incubated with His-PP1α or His-PP1γ for the indicated time points and immunoblotted for pS674/pS684 and Kif18A. Coomassie staining (CBB) showing purified PP1. Immunoblots showing the specificity of the pS674 and pS684 antibodies are shown inSupplementary Fig. 1c. Figure 3: PP1α and PP1γ dephosphorylate Kif18A at S674 and S684. ( a ) GFP and Kif18A immunoblots of input samples, supernatant (SN), and GFP immunoprecipitates (IP) from mitotic (nocodazole release in MG132) cells transfected with GFP, GFP-PP1α or GFP-PP1γ. Asterisk indicates unspecific band. A long exposure of the GFP immunoblot is shown in Supplementary Fig. 1g . ( b ) and ( c ) In vitro pull-down assays using WT, PP1-binding deficient (PP1Δ), non-phosphorylatable (2A), and double defective (PP1Δ+2A) GST-Kif18A CT . Kif18A and PP1 immunoblots showing input and bead bound GST-Kif18A CT associated with His-PP1α ( b ) or His-PP1γ ( c ). ( d ) Experimental outline of in vitro PP1 phosphatase assays: GST-Kif18A CT was prephosphorylated by incubation with Cdk1/cyclin B1 and the PP1 isoforms or buffer control were added to the kinase reaction without removing Cdk1/cyclin B1. ( e ) and ( f ) In vitro Cdk1/cyclin B1 phosphorylated WT ( e ) and PP1 binding deficient (PP1Δ) ( f ) GST-Kif18A CT were incubated with His-PP1α or His-PP1γ for the indicated time points and immunoblotted for pS674/pS684 and Kif18A. Coomassie staining (CBB) showing purified PP1. Immunoblots showing the specificity of the pS674 and pS684 antibodies are shown in Supplementary Fig. 1c . Full size image PP1 antagonizes Cdk1’s effect on Kif18A If PP1-mediated dephosphorylation of Kif18A is critical for its function, a mutant resistant to dephosphorylation should cause a plate thinning phenotype contrary to that of non-phosphorylatable GFP-Kif18A 2A . Unfortunately, the expression of the phosphomimetic mutant (Kif18A 2D , S674D/S684D) in Kif18A-RNAi cells had no effect on either the timing of plate thinning or final plate width ( Supplementary Fig. 1d,e ) suggesting that the introduced negative charges did not functionally mimic phosphorylated S674/S684. Therefore, we monitored chromosome movements in Kif18A-RNAi cells expressing GFP-Kif18A PP1Δ deficient in PP1-mediated dephosphorylation ( Fig. 4a and Supplementary Movie 4 ). Consistent with the observation that S674/S684 phosphorylation did not affect chromosome congression, all three cell lines—Kif18A-RNAi cells expressing either GFP-Kif18A WT , -Kif18A 2A or -Kif18A PP1Δ —were equally efficient in chromosome alignment ( Fig. 4b ). As shown before ( Fig. 2d,e ), GFP-Kif18A 2A induced metaphase plate thinning prematurely ( Fig. 4b ). Notably, metaphase plate thinning was also observed in cells expressing GFP-Kif18A PP1Δ , but the plates that finally formed were significantly broader compared with control cells ( Fig. 4b,c ). Measurement of sister kinetochore distance revealed that this increase in metaphase plate width was not mediated by an increased stretching of sister KTs ( Supplementary Fig. 1h ) indicating that GFP-Kif18A PP1Δ expressing cells indeed fail to tightly align their chromosomes at the spindle equator. 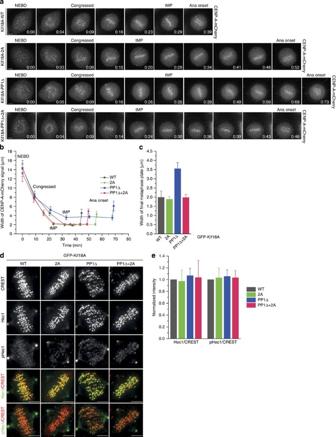Figure 4: Cells expressing Kif18APP1Δdisplay broader metaphase plates. (a) Still images showing Kif18A-RNAi cells inducibly expressing WT, 2A, PP1Δ and PP1Δ+2A GFP-Kif18A. CENP-A-mCherry was used to monitor KT movements. Time stamp at NEBD was set to 0:00 minutes. Scale bar, 5.6 μm. See alsoSupplementary Movie 4. (b) Diagram illustrating the changes in width of the CENP-A-mCherry signal over time at indicated time points. Points represent mean±s.d. from five independent experiments withn=94 cells for WT,n=115 cells for 2A,n=75 cells for PP1Δ andn=85 cells for PP1Δ+2A. (c) Quantification of the final width of the metaphase plate from cells analysed inb. Bar graphs show mean±s.d. See alsoSupplementary Fig. 1h. (d) Immunofluorescence images of Kif18A-RNAi cells expressing the indicated GFP-Kif18A variants and arrested in mitosis by MG132 treatment. Cells were fixed and immunostained for Hec1, phospho-Hec1 (pS55, pHec1) and CREST. Images are maximum intensity projections of deconvolvedz-stacks. Scale bar, 4 μm. (e) Hec1 and pHec1 intensities were set relative to total CREST levels and normalized to Hec1/CREST and pHec1/CREST ratio of WT GFP-Kif18A. Bar graphs show the mean±s.d. from three independent experiments with more than 40 cells per condition. Figure 4: Cells expressing Kif18A PP1Δ display broader metaphase plates. ( a ) Still images showing Kif18A-RNAi cells inducibly expressing WT, 2A, PP1Δ and PP1Δ+2A GFP-Kif18A. CENP-A-mCherry was used to monitor KT movements. Time stamp at NEBD was set to 0:00 minutes. Scale bar, 5.6 μm. See also Supplementary Movie 4 . ( b ) Diagram illustrating the changes in width of the CENP-A-mCherry signal over time at indicated time points. Points represent mean±s.d. from five independent experiments with n =94 cells for WT, n =115 cells for 2A, n =75 cells for PP1Δ and n =85 cells for PP1Δ+2A. ( c ) Quantification of the final width of the metaphase plate from cells analysed in b . Bar graphs show mean±s.d. See also Supplementary Fig. 1h . ( d ) Immunofluorescence images of Kif18A-RNAi cells expressing the indicated GFP-Kif18A variants and arrested in mitosis by MG132 treatment. Cells were fixed and immunostained for Hec1, phospho-Hec1 (pS55, pHec1) and CREST. Images are maximum intensity projections of deconvolved z -stacks. Scale bar, 4 μm. ( e ) Hec1 and pHec1 intensities were set relative to total CREST levels and normalized to Hec1/CREST and pHec1/CREST ratio of WT GFP-Kif18A. Bar graphs show the mean±s.d. from three independent experiments with more than 40 cells per condition. Full size image Next, we sought to confirm that the GFP-Kif18A PP1Δ phenotype was indeed due to a failure of S674/S684 dephosphorylation. Unfortunately, we were unable to determine phosphorylation levels of Kif18A by immunofluorescence microscopy as the pS674/pS684 Kif18A antibodies failed to detect Kif18A under all fixation conditions tested. Thus, to test if hyperphosphorylated Kif18A accounts for the observed phenotype, we introduced the 2A mutation in GFP-Kif18A PP1Δ and analysed if these non-phosphorylatable mutations abrogate the Kif18A PP1Δ phenotype. And indeed, Kif18A-RNAi cells expressing GFP-Kif18A PP1Δ+2A behaved like the 2A-expressing cells: they prematurely initiated metaphase plate thinning and the final widths of the thinnest plates were comparable to the ones in WT-expressing cells ( Fig. 4b,c ). To further confirm that the interaction between PP1 and Kif18A is critical for the dephosphorylation of Kif18A rather than for the transport of PP1 to KTs, we analysed Hec1, a KT component whose phosphorylation state is highly sensitive to the activities of Aurora-B and PP1 at KTs [26] , [27] . Phospho-specific antibodies demonstrated that expression of GFP-Kif18A PP1Δ in Kif18A-RNAi cells did not affect the phosphorylation levels of Hec1 at KTs ( Fig. 4d,e ) suggesting that Kif18A does not contribute to the bulk KT localization of PP1. In conclusion, this series of experiments strongly supports our hypothesis that dephosphorylation of Kif18A by PP1 is critical for proper plate thinning as cells progress towards anaphase. GFP-Kif18A 2A suppresses chromosome oscillations Reportedly, Kif18A limits the oscillation amplitude of chromosomes by reducing their oscillation speed [4] , [12] . Therefore, our data suggest that chromosomes in GFP-Kif18A 2A -expressing cells display decreased chromosome velocity, whereas PP1Δ expression should increase the oscillation speed. To quantify the oscillatory movements of chromosomes, we applied a previously established method that determines the deviation of average position (DAP) for individual KTs as a linear measure of oscillation amplitude [12] . In WT-expressing Kif18A-RNAi cells, the DAP was 0.41±0.16 μm ( Fig. 5b and Supplementary Movie 5 ), which was in agreement with previously published data (DAP of 0.46±0.02 μm (ref. 12 )). And indeed, the expression of GFP-Kif18A 2A significantly reduced the DAP to 0.27±0.10 μm and this effect was mediated by a reduction in the oscillation speed from 1.87±0.75 μm min −1 in WT-expressing cells to 1.36±0.71 μm min −1 in 2A GFP-Kif18A expressing cells ( Fig. 5a–c and Supplementary Movie 5 ). In contrast, GFP-Kif18A PP1Δ increased the oscillation speed resulting in an elevated DAP of 0.59±0.18 μm ( Fig. 5a–c and Supplementary Movie 5 ). Consistent with the plate thinning phenotype ( Fig. 4b,c ), introducing the 2A mutation (GFP-Kif18A PP1Δ+2A ) abrogated the hyperoscillation phenotype. Collectively, these data suggest that Cdk1 phosphorylation of Kif18A at S674/S684 negatively affects the ability of Kif18A to suppress the oscillation amplitude of bioriented chromosomes. 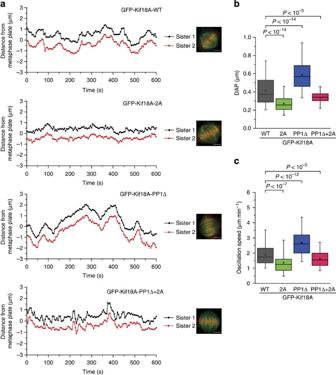Figure 5: Phosphorylation of Kif18A at S674/S684 influences KT oscillation. (a) Distance versus time plots showing KT oscillation around the metaphase plate (MP). Shown is the movement of a single sister-KT-pair for Kif18A-RNAi cells expressing WT, non-phosphorylatable (2A), PP1-binding deficient (PP1Δ) or double defective (PP1Δ+2A) GFP-Kif18A. Two-colour images of GFP-Kif18A (green) and CENP-A-mCherry (red) were taken immediately after imaging of KT-movement was stopped. Scale bar, 4 μm. See alsoSupplementary Movie 5. (b) and (c) Quantification of DAP as measurement for the oscillation amplitude (b) and oscillation speed (c) for single KTs. Box plots show 5th, 95th (whiskers) and 25th, 50th, 75th percentile (boxes). Square represents mean. More than 50 sister KT pairs from 9 to 11 cells per condition were plotted from at least four independent experiments. Statistical difference was determined by a two-tailed, unpaired Student’st-test. Figure 5: Phosphorylation of Kif18A at S674/S684 influences KT oscillation. ( a ) Distance versus time plots showing KT oscillation around the metaphase plate (MP). Shown is the movement of a single sister-KT-pair for Kif18A-RNAi cells expressing WT, non-phosphorylatable (2A), PP1-binding deficient (PP1Δ) or double defective (PP1Δ+2A) GFP-Kif18A. Two-colour images of GFP-Kif18A (green) and CENP-A-mCherry (red) were taken immediately after imaging of KT-movement was stopped. Scale bar, 4 μm. See also Supplementary Movie 5 . ( b ) and ( c ) Quantification of DAP as measurement for the oscillation amplitude ( b ) and oscillation speed ( c ) for single KTs. Box plots show 5th, 95th (whiskers) and 25th, 50th, 75th percentile (boxes). Square represents mean. More than 50 sister KT pairs from 9 to 11 cells per condition were plotted from at least four independent experiments. Statistical difference was determined by a two-tailed, unpaired Student’s t -test. Full size image S674/S684 phosphorylation affects Kif18A localization We next investigated how S674/S684 phosphorylation affects the function of Kif18A. Since Kif18A’s ability to suppress chromosome movements depends on its KT-MT plus-end accumulation [10] , [13] , [15] , we investigated if S674/S684 phosphorylation affects the localization of Kif18A. Indeed, while GFP-Kif18A WT expressed in mitotically arrested Kif18A-RNAi cells efficiently accumulated at the plus-ends of kinetochore MTs, GFP-Kif18A PP1Δ prominently decorated their lattice ( Fig. 6a–c ). Importantly, this defect was mediated by S674/S684 phosphorylation as double-deficient Kif18A (GFP-Kif18A PP1Δ+2A ) localized normally ( Fig. 6a–c ). Consistent with the observation that Kif18A 2A affects the timing of plate thinning but not the final plate width, GFP-Kif18A 2A localized normally under these conditions where cells were arrested in late metaphase by MG132 treatment ( Fig. 6a–c ). To resolve the temporal difference in plus-end localization of Kif18A WT and Kif18A 2A , we performed live-cell analysis. Upon chromosome congression, GFP-Kif18A WT displayed prominent lattice localization before it gradually accumulated at MT plus-ends ( Fig. 6d,e and Supplementary Movie 6 ). Intriguingly, GFP-Kif18A 2A was able to accumulate at MT plus-ends significantly earlier than WT-Kif18A ( Fig. 6d,e and Supplementary Movie 7 ) indicating that S674/S684 phosphorylation interferes with Kif18A localization. 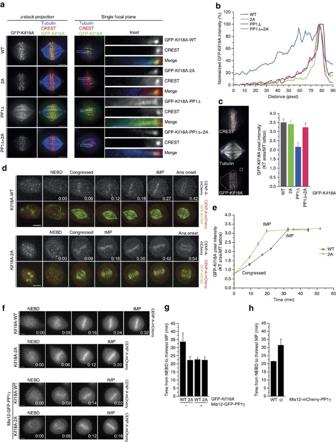Figure 6: S674/S684 phosphorylation affects Kif18A localization. (a) Immunofluorescence images showing the localization of GFP-Kif18A variants in MG132-treated Kif18A-RNAi cells. Cells were fixed and stained for alpha-tubulin and CREST. Images are maximum intensity projections of deconvolvedz-stacks (left). Insets from a single focal plane represent the localization of the GFP-Kif18A variants along a selected K-fibre (right). Scale bar, 4 μm. (b) Linescan over a 1-pixel-window showing the normalized intensity of GFP-Kif18A variants from insets shown ina. (c) Quantification ofarepresenting the ratio of GFP-Kif18A localization at KTs (KT area) versus the microtubule lattice (MT lattice). Bar graphs represent the mean±s.d. from at least four independent experiments with more than 90 cells. (d) Time-lapse images showing the dynamic localization of WT or 2A GFP-Kif18A over time in Kif18A-RNAi cells. Co-expression of CENP-A-mCherry was used to determine mitotic timing. Indicated are the time points according to the categories described inFig. 2c. Time stamp at NEBD was set to 0:00 minutes. Scale bar, 4 μm. See alsoSupplementary Movies 6 and 7. (e) Quantification ofdshowing the GFP-Kif18A plus-tip accumulation over time as ratio of Kif18A at the KT area versus microtubule lattice. Points represent mean±s.d. from two independent experiments withn=26 cells (WT) orn=39 cells (2A). (f) Still images of movies showing HeLa cells stably expressing CENP-A-mCherry and inducibly expressing WT or 2A GFP-Kif18A transiently transfected with Mis12-GFP-PP1γ. Time stamp at NEBD was set to 0:00 minutes. Scale bar, 5.6 μm. See alsoSupplementary Movie 9. (g) Quantification of the time to form a tMP from cells shown inf. Bars show mean±s.d. from four independent experiments withn=27 and 50 cells (WT±Mis12-GFP-PP1γ) orn=51 and 43 cells (2A±Mis12-GFP-PP1γ). (h) Quantification of MP thinning in cells inducibly expressing WT or catalytic inactive versions (ci, D64N) of Mis12-mCherry-PP1γ. Bar graphs represent mean from two independent experiments withn=56 cells for WT andn=50 cells for ci. Error bars show s.d. Figure 6: S674/S684 phosphorylation affects Kif18A localization. ( a ) Immunofluorescence images showing the localization of GFP-Kif18A variants in MG132-treated Kif18A-RNAi cells. Cells were fixed and stained for alpha-tubulin and CREST. Images are maximum intensity projections of deconvolved z -stacks (left). Insets from a single focal plane represent the localization of the GFP-Kif18A variants along a selected K-fibre (right). Scale bar, 4 μm. ( b ) Linescan over a 1-pixel-window showing the normalized intensity of GFP-Kif18A variants from insets shown in a . ( c ) Quantification of a representing the ratio of GFP-Kif18A localization at KTs (KT area) versus the microtubule lattice (MT lattice). Bar graphs represent the mean±s.d. from at least four independent experiments with more than 90 cells. ( d ) Time-lapse images showing the dynamic localization of WT or 2A GFP-Kif18A over time in Kif18A-RNAi cells. Co-expression of CENP-A-mCherry was used to determine mitotic timing. Indicated are the time points according to the categories described in Fig. 2c . Time stamp at NEBD was set to 0:00 minutes. Scale bar, 4 μm. See also Supplementary Movies 6 and 7 . ( e ) Quantification of d showing the GFP-Kif18A plus-tip accumulation over time as ratio of Kif18A at the KT area versus microtubule lattice. Points represent mean±s.d. from two independent experiments with n =26 cells (WT) or n =39 cells (2A). ( f ) Still images of movies showing HeLa cells stably expressing CENP-A-mCherry and inducibly expressing WT or 2A GFP-Kif18A transiently transfected with Mis12-GFP-PP1γ. Time stamp at NEBD was set to 0:00 minutes. Scale bar, 5.6 μm. See also Supplementary Movie 9 . ( g ) Quantification of the time to form a tMP from cells shown in f . Bars show mean±s.d. from four independent experiments with n =27 and 50 cells (WT±Mis12-GFP-PP1γ) or n =51 and 43 cells (2A±Mis12-GFP-PP1γ). ( h ) Quantification of MP thinning in cells inducibly expressing WT or catalytic inactive versions (ci, D64N) of Mis12-mCherry-PP1γ. Bar graphs represent mean from two independent experiments with n =56 cells for WT and n =50 cells for ci. Error bars show s.d. Full size image Our data presented so far indicate that PP1-dependent dephosphorylation of S674/S684 induces Kif18A-mediated plate thinning. Reportedly, recruitment of PP1 to outer KTs is negatively regulated by Aurora-B-mediated phosphorylation of KNL1 and, accordingly, their physical separation on chromosome biorientation facilitates KT localization of PP1 (refs 18 , 28 , 29 , 30 ). On the basis of these observations, we speculated that uncoupling KT localization of PP1 from chromosome biorientation should cause premature plate thinning. To test this, the timing of plate thinning was analysed in cells where PP1 was constitutively targeted to KTs by fusion to the outer KT protein Mis12. Time-lapse analyses confirmed that Mis12-GFP-PP1γ localized prematurely in prophase to KTs ( Supplementary Fig. 2a and Supplementary Movie 8 ). Strikingly, expression of Mis12-GFP-PP1γ enabled Kif18A WT -expressing cells to establish a thin plate with the same timing as 2A-expressing cells ( Fig. 6f,g and Supplementary Movie 9 ). Expression of Mis12-GFP-PP1γ did not accelerate thin plate formation in GFP-Kif18A 2A -expressing cells suggesting that the effect of Mis12-GFP-PP1γ on plate thinning is mediated via S674/S684 dephosphorylation ( Fig. 6f,g and Supplementary Movie 9 ). Consequently, targeting catalytic inactive PP1γ D64N (Mis12-GFP-PP1γ ci ) (ref. 31 [31] ) had no effect on the timing of thinnest plate formation ( Fig. 6h ). Thus, these data strongly support our model that PP1 dephosphorylation of Kif18A triggers metaphase plate thinning. Altered chromosome oscillations result in segregation errors Finally, we investigated how deregulated plate thinning impairs the fidelity of chromosome segregation. To this end, thymidine presynchronized Kif18A-RNAi cells expressing GFP-Kif18A WT , -Kif18A 2A , -Kif18A PP1Δ or Kif18A PP1Δ+2A were treated with the Eg5 inhibitor VS-83 (ref. 32 ) to induce monopolar spindle formation and following VS-83 washout cells were processed for immunofluorescence analyses. As reported previously [33] , transient Eg5 inhibition causes a drastic increase in the incidence of erroneous chromosome segregation events allowing us to monitor the fidelity of sister chromatid segregation under stringent conditions. Importantly, Kif18A-RNAi cells expressing either non-phosphorylatable (2A), GFP-Kif18A (PP1Δ) deficient in PP1 dephosphorylation or the GFP-Kif18A double mutant (PP1Δ+2A) had significantly more defects in chromosome segregation than identically treated GFP-Kif18A WT -expressing cells. Thus, these data demonstrate that timely controlled plate thinning is central for the maintenance of genome stability in tissue culture cells. Upon congression, vertebrate chromosomes display rapid oscillatory movements [34] , [35] and, as previously suggested, these oscillations facilitate the alignment of chromosomes and protects them from becoming entangled [5] . Consistent with previous reports [1] , [4] , [36] , our live-cell analyses revealed that the width of the metaphase plate significantly decreased upon chromosome congression in HeLa-, RPE1- and LLC-PK1 but not in Ptk2-cells ( Supplementary Fig. 2b–d ) suggesting that higher mammalian cells prepare for sister chromatid segregation by reducing the oscillatory movements of chromosomes resulting in the tight alignment of all chromosomes at the spindle equator shortly before anaphase onset. Our data establish that Cdk1 and PP1 antagonistically control chromosome oscillations via Kif18A. Specifically, our data indicate that in early metaphase, Cdk1 promotes chromosome oscillations by interfering with efficient plus-end accumulation of Kif18A. How does Cdk1 prevent plus-end accumulation of Kif18A? In vitro motility assays revealed that Cdk1 phosphorylation did not affect the velocity of full-length His-GFP-Kif18A WT ( Supplementary Fig. 2f–h ) leaving the possibility that Cdk1 prevents plus-end accumulation of Kif18A by decreasing its processivity and/or MT plus-end pausing time. Unfortunately, the conditions of the in vitro kinase and total internal reflection fluorescence microscopy assays were not compatible with each other and since the phosphomimetic mutations (S674D/S684D) did not functionally mimic phosphorylation ( Supplementary Fig. 1d,e ), we were unable to determine if S674/S684 phosphorylation affects Kif18A’s processivity and/or plus-end pausing time. Thus, exactly how Cdk1 affects the plus-end accumulation of Kif18A is an open question that merits further investigation. The inhibitory effect of Cdk1 on Kif18A is released by PP1 that directly dephosphorylates Kif18A at S674/S684. Thus, our study revealed that PP1 not only stabilizes MT attachment by dephosphorylating Aurora-B substrates at KTs [18] , [28] , [29] , [30] but also induces plate thinning by dephosphorylating Kif18A. At the same time, this finding establishes Kif18A as the first Cdk1 substrate—apart from PP1 itself [37] , [38] , [39] —that is directly dephosphorylated by PP1 demonstrating that PP1 can act as an antagonist of not only Aurora-B but also Cdk1. Dephosphorylation of Kif18A by PP1 depends on a conserved PP1-binding motif located in the C-terminus of Kif18A ( Fig. 3b,c ). The presence of a PP1-binding motif raises the question of whether Kif18A functions as a transport molecule to deliver PP1 to KTs. However, this seems unlikely because the phosphorylation levels of Hec1—which are highly sensitive to Aurora-B and PP1 activities at KTs [26] , [27] —were not affected by replacing endogenous Kif18A with GFP-Kif18A PP1Δ . Furthermore, fluorescence recovery after photobleaching experiments revealed that the dynamic localization of PP1 to KTs was not altered by nocodazole-induced MT depolymerization [40] , a condition that prevents Kif18A from localizing to KTs. Thus, Kif18A does not significantly contribute to the KT localization of PP1 which as shown previously is primarily mediated by KNL1 (ref. 18 ) and to a lesser extent by Sds22 (ref. 29 ) and CENP-E [28] . Notably, an interaction between Kinesin-8 and PP1 has been recently reported for fission yeast Klp5/Klp6 and this interaction has been shown to be essential for timely SAC silencing [25] . Our data revealed that the expression of Kif18A deficient in PP1 binding (GFP-Kif18A PP1Δ ) as well causes a delay in anaphase onset ( Fig. 4b ) suggesting that human Kif18A might also play a role in SAC silencing. However, the delay in anaphase onset was attenuated by introducing the 2A mutation into PP1-binding deficient Kif18A (GFP-Kif18A PP1Δ+2A ; Fig. 4b ) indicating that the mitotic defect of Kif18A PP1Δ might be primarily due to deregulated Kif18A itself. Thus, while we cannot formally exclude the possibility that Kif18A might play an additional role in SAC silencing, all our current data indicate that PP1 binding to Kif18A is critical for dephosphorylation of S674/S684 and, hence, for the timely onset of metaphase plate thinning in pre-anaphase cells. The importance of PP1 binding for Kif18A function raises the question of when during spindle assembly the two proteins interact. One scenario could be that PP1 constitutively interacts with Kif18A, that is, Kif18A brings along its own phosphatase as it moves towards the plus-ends of MTs. However, if this applies, it is difficult to reconcile why artificial targeting of PP1γ to KTs (Mis12-GFP-PP1γ) in cells that express WT-Kif18A induces premature formation of a tMP ( Fig. 6g ) and why this effect depends on the catalytic activity of KT-targeted PP1γ ( Fig. 6h ). Since Mis12-GFP-PP1γ does not further accelerate plate thinning in GFP-Kif18A 2A -expressing cells, these data indicate that the effect of Mis12-GFP-PP1γ on the timing of plate thinning is mediated via Kif18A dephosphorylation. Thus, based on these data, we favour a scenario where KT-recruited PP1 binds to Kif18A as it approaches the plus-ends of KT-MTs. Specifically, we propose the following model ( Fig. 7d–f ): In early metaphase, Cdk1-mediated phosphorylation of Kif18A at S674/S684 prevents it from efficiently accumulating at the plus-ends of KT-MTs. Since plus-end localization is a prerequisite for Kif18A’s inhibitory effect on the oscillation amplitude, chromosomes during early metaphase display vigorous motions around the spindle equator. At that time in mitosis, centromere tension is low allowing the inner centromere kinase Aurora-B to prevent PP1 from being efficiently recruited to KTs by phosphorylating the outer KT protein KNL1 at its PP1-binding motif RVSF [18] . As the KT attachment of bioriented chromosomes matures and forces acting on sister KTs increase, Aurora-B and KNL1 spatially separate resulting in the recruitment of PP1 to outer KTs. By dephosphorylating Aurora-B substrates, PP1 further promotes the stabilization of KT-MT attachments, which induces SAC silencing and APC/C activation. As the activity of Cdk1 declines, the balance tips in favour of PP1-mediated dephosphorylation of S674/S684 resulting in efficient plus-end accumulation of Kif18A and, hence, in suppressed chromosome oscillations. Thus, our model implies that cells by coupling the phosphorylation state of Kif18A to the attachment state of chromosomes are able to maintain chromosome oscillations when they are beneficial, that is, during the initial phase of chromosome alignment and, subsequently, to dampen them to ensure the tight positioning of chromosomes at the metaphase plate. And indeed, interfering with this regulatory mechanism by replacing endogenous Kif18A with Kif18A deficient in either Cdk1 phosphorylation (2A), in PP1-mediated dephosphorylation (PP1Δ) or both (PP1Δ+2A) caused a drastic increase in the rate of chromosome segregation defects ( Fig. 7a–c ). Thus, these data suggest that timely controlled chromosome dynamics in pre-anaphase cells are important for the maintenance of genome stability. Given this central function, it is conceivable that additional factors might exist that control chromosome dynamics in a manner that depends as well on the antagonistic activities of Cdk1 and PP1. Clearly, future studies are required to identify these potential factors and to dissect how their activities are coordinated with the function of Kif18A to ensure that the dynamic behaviour of chromosomes is precisely adjusted to the different requirements of distinct pre-anaphase stages. 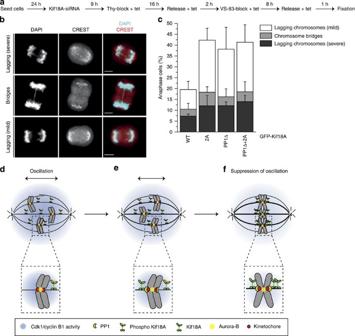Figure 7: Altered chromosome oscillations result in segregation errors. (a) Experimental outline of VS-83-release under Kif18A-rescue conditions. (b) Immunofluorescences images of anaphase cells with segregation defects. After VS-83-release, cells were fixed and stained for CREST and Hoechst. A single focal plane of deconvolved images is shown. Scale bar, 5.6 μm. (c) Quantification of segregation errors in anaphase cells fromb, which were depleted of endogenous Kif18A and express GFP-Kif18A variants. Bars represent mean±s.d. from four independent experiments with more than 120 cells per condition. (d) During prometaphase, interkinetochore tension is low enabling Aurora-B to prevent PP1 localization by phosphorylating KNL1. Cdk1 phosphorylation of Kif18A prevents it from efficiently accumulating at the plus-tips of KT-MTs. (e) APC/C-mediated cyclin B1 destruction initiates at metaphase resulting in decreasing Cdk1 activity. Concurrently, PP1 starts to accumulate at outer KTs as chromosomes achieve biorientation. This results in a local dephosphorylation of Kif18A and a gradual suppression of chromosome oscillations. (f) In late metaphase, the balance is tipped in favour of dephosphorylated Kif18A resulting in reduced oscillation amplitude with chromosomes tightly aligned at the spindle equator. Figure 7: Altered chromosome oscillations result in segregation errors. ( a ) Experimental outline of VS-83-release under Kif18A-rescue conditions. ( b ) Immunofluorescences images of anaphase cells with segregation defects. After VS-83-release, cells were fixed and stained for CREST and Hoechst. A single focal plane of deconvolved images is shown. Scale bar, 5.6 μm. ( c ) Quantification of segregation errors in anaphase cells from b , which were depleted of endogenous Kif18A and express GFP-Kif18A variants. Bars represent mean±s.d. from four independent experiments with more than 120 cells per condition. ( d ) During prometaphase, interkinetochore tension is low enabling Aurora-B to prevent PP1 localization by phosphorylating KNL1. Cdk1 phosphorylation of Kif18A prevents it from efficiently accumulating at the plus-tips of KT-MTs. ( e ) APC/C-mediated cyclin B1 destruction initiates at metaphase resulting in decreasing Cdk1 activity. Concurrently, PP1 starts to accumulate at outer KTs as chromosomes achieve biorientation. This results in a local dephosphorylation of Kif18A and a gradual suppression of chromosome oscillations. ( f ) In late metaphase, the balance is tipped in favour of dephosphorylated Kif18A resulting in reduced oscillation amplitude with chromosomes tightly aligned at the spindle equator. Full size image Cell culture HeLa cells were obtained from ATCC and cultured as described [41] . HeLa cell lines stably expressing CENP-A-mCherry were generated by random integration according to the manufacturer’s (Invitrogen) instructions. Stable CENP-A-mCherry-expressing clones were used for integration of GFP-Kif18A variants or GFP-cyclin B1 at a predefined genomic FRT (flippase (Flp) recognition target). Expression of GFP-cyclin B1, GFP-Kif18A variants or Mis12-mCherry-PP1γ were induced by addition of 0.1 μg ml −1 , 2 μg ml −1 or 5 μg ml −1 Tetracycline hydrochloride (Sigma), respectively. siRNA transfections Cells (30,000–40,000 ml −1 ) were seeded and siRNA transfections were performed using Oligofectamine (Invitrogen) and the following siRNA oligonucleotides (Thermo Scientific) at 75 nM final concentration: luciferase Gl2, Kif18A and Mad2 (ref. 24 ). Cells were processed for immunofluorescence or lysed for immunoblotting. For depletion of cyclin A2, 100,000 cells ml −1 were seeded and after 6 h transfected with cyclin A2 siRNA [42] at 25 or 50 nM final concentration using Oligofectamine (Invitrogen). Twenty-four hours after transfection, cells were blocked in 2 mM thymidine for 20 h. Transfection experiments Cells (100,000–200,000 ml −1 ) were seeded and grown for 24 h before transfection. HeLa cells stably expressing CENP-A-mCherry and inducibly expressing GFP-Kif18A were transfected with mCherry-cyclin B1 ( Fig. 2f,g ) or Mis12-GFP-PP1γ ( Fig. 6f,g and Supplementary Fig. 2a ) using X-treme-Gene-9 DNA Transfection Reagent (Roche) in a 3:1 ratio. Cells were synchronized by a single thymidine block. For co-immunoprecipitation experiments ( Fig. 3a ), 5 × 10 6 cells were seeded and 24 h later transfected according to manufacturer’s protocol using X-treme-Gene-9 DNA Transfection Reagent. Live-cell microscopy HeLa cells stably expressing CENP-A-mCherry and inducible GFP-Kif18A variants were seeded into μ-slide 8 well (Ibidi). For Fig. 5 , a media exchange was performed instead of a thymidine block and for co-depletion of Mad2 ( Supplementary Fig. 1f ) Mad2-siRNA was added together with Kif18A-siRNA. For the analysis of metaphase plate thinning in different cell lines ( Supplementary Fig. 2b–e ), 1.5 × 10 5 cells ml −1 were seeded in 5 mM thymidine for 21 h and imaged 9 h after release. For imaging, CO 2 -independent (Gibco) live cell media supplemented with 10% FCS (Invitrogen), 100 U ml −1 penicillin, 100 μg ml −1 streptomycin (Gibco) and 1 × GlutaMAX (Invitrogen) was used. Cells were imaged at 37 °C using DeltaVision-Core system (Applied Precision) mounted on a IX-71 inverted microscope (Olympus) equipped with an environmental chamber, Arc-lamp and a CoolSnap-HQ-2 camera (Photometrics). Before time-lapse imaging, a single image was acquired in the fluoresceinisothiocyanate (FITC) and tetramethylrhodamine isothiocyanate (TRITC) channel to determine the expression level of GFP-Kif18A. To record mitotic timing, a 40 × 1.35 NA UApo/340 (Olympus) oil objective was used and a single focal plane in the TRITC and/or FITC channel for 12 h duration was acquired. To record KT oscillations ( Fig. 5 ), cells were imaged using a 100 × 1.40 NA UPLS Apo (Olympus) oil objective. Five image planes with 0.5 μm z -stack size were acquired at 5 s time interval for 10 min duration in the TRITC channel. Afterwards, images for FITC and TRITC channel with 0.5 μm spacing over the range of the CENP-A-signal were acquired. Plus-end localization of GFP-Kif18A ( Fig. 6d ) over time was analysed using a spinning-disk confocal microscope (Axio Observer Z1) equipped with an environmental chamber (Zeiss), a 488 nm OPLS and a 561 nm Diode laser. Cells were imaged at 37 °C using a 63 × 1.4 NA Plan Apochromat (Zeiss) oil objective. Single z -stack sections were acquired at 3 min time intervals for 12 h duration. Cells in Supplementary Fig. 1d–f were imaged at 37 °C using a 20 × 0.4 NA LD Plan Neo (Zeiss) objective on a Axio Observer Z1 (Zeiss) equipped with Colibri-LED-modules and a CoolSnap-ES2 camera (Photometrics). Images were acquired at 4 min time interval for 12 h duration. Immunofluorescence microscopy Cells were seeded on coverslips and 9 h after thymidine-release, 20 μM MG132 was added for 1 h. For the analysis of segregation defects, the experimental setup shown in Fig. 7a was used. For phospho-Hec1 staining, cells were permeabilized for 2 min at 37 °C (60 mM Pipes, 25 mM Hepes, 10 mM EGTA and 2 mM MgCl 2 , pH 7.0) and 0.2% TX-100 and then fixed for 2 × 5 min at 37 °C in pre-warmed PHEM-buffer and 3.7% formaldehyde. During permeabilization, fixation and blocking phosphatase inhibitors (20 mM β-Glycerophosphate, 20 mM NaF, 0.3 mM NaV) were included. For all other stainings, cells were permeabilized and fixed for 12 min at room temperature (RT) in 100 mM Pipes pH 6.8, 10 mM EGTA, 1 mM MgCl 2 , 0.2% TX-100 and 3.7% formaldehyde. Cells were washed with TBS-T (TBS +0.1% TX-100) and blocked overnight at 4 °C in blocking-buffer (2% BSA, 0.02% Azid in TBS-T). Primary antibodies diluted in blocking-buffer were added and incubated for 1 h at RT. Cells were washed 3 × 10 min with TBS-T and then incubated with secondary antibodies diluted in blocking-buffer for 1 h at RT. After washing 3 × 10 min with TBS-T, coverslips were mounted onto glass slides in Mowiol (4–88, Polysciences) mounting-medium. Images were acquired using the DeltaVision-Core system described above. For imaging, a 100 × 1.40 NA UPLS Apo oil objective (Olympus) was used and z -stacks with 0.2 μm distance were recorded. For the imaging of the segregation defects ( Fig. 7b,c ), a 40 × 1.35 NA UApo/340 (Olympus) oil objective was used and z -stacks with 0.5 μm distance were recorded. For immunofluorescence staining, the following antibodies were used: CREST serum (1:2,000; Immunovision); anti-human Hec1 (1:500; GeneTex, GTX70268); anti-human phospho-S55 Hec1 (1:300; GeneTex, GTX70017); anti-human DM1α-tubulin (1:1,000–1:2,000; Sigma, T6199); anti-mouse alpha-tubulin (1:100; AA4.3, hypridoma supernatant in 1% FCS); Hoechst H33342 (1:3,000; Sigma); anti-human alexa fluor 568 (1:1,000; Invitrogen, A21090); anti-mouse alexa fluor 350 (1:50; Invitrogen, A11045). anti-rabbit alexa fluor 647 (1:1,000; Invitrogen, A21245). Image processing and quantification Images were taken at identical exposure times within each experiment, acquired as 16-bit images, deconvolved using SoftWorx 4.0 software (Applied Precision) and quantified with ImageJ (NIH). Stable co-expression of CENP-A-mCherry was used to determine the timing between NEBD and congression of chromosomes to the metaphase plate (Congressed), from congression to the establishment of a tMP, and from the formation of a tMP to anaphase onset (Ana onset). The width of the CENP-A-mCherry signal was measured as illustrated in Supplementary Fig. 1a . NEBD, congressed, tMP and anaphase onset (Ana onset) were used as defined time points from the analysis of the mitotic timing. For measuring the decay of cyclin B1 intensities a circular region with fixed diameter was centred on each cell and the raw integrated intensity was measured over the entire movie. Intensity values were corrected for background signal and normalized to values at NEBD. In fixed samples, the interkinetochore distance was measured for five sister KT pairs in single focal planes and the mean for each cell was calculated. Cells in which the spindle was tilted, visible by appearance of spindle poles in different z -stack planes, were excluded from the analysis. To analyse the Kif18A localization pattern on maximum intensity projections ( Fig. 6c ), first a polygon selection covering all KTs (CREST-signal) for Kif18A localization at the KT area and second a polygon selection around the microtubule lattice (tubulin-signal) for Kif18A lattice localization was drawn. Image raw integrated intensities were measured, divided by the corresponding area-size and corrected for the background signal (white square). The ratio of Kif18A pixel intensity at KT area versus MT lattice was calculated. To analyse the Hec1 and phospho-Hec1 levels ( Fig. 4e ), image raw integrated intensities were measured (using the ImageJ multi-measure Plug-in) over the total z-stack plane using a polygon selection covering all KTs of the mitotic spindle. Measurements were performed for all three channels at the same position. The measured intensity was divided by the area of the selection and the background was subtracted. Afterwards the mean of the signal intensity over all z-stacks was calculated and the ratio of the signal of interest to CREST was determined and normalized to the ratio of cells expressing GFP-Kif18A WT. KT movements ( Fig. 5 ) were manually tracked in one of the five single z-stack planes using MTrackJ plug-in for ImageJ. Quantification of DAP was performed for each KT separately as previously described [12] . Oscillation speed was quantified as the total distance a kinetochore moved divided by the time the kinetochore was filmed. Movement in z-direction was avoided as movement of sister kinetochore pairs was only tracked in single focal planes (0.5 μm). Cells with rotating or rocking spindles identified by identical vectorial movements of multiple KTs were excluded from the analyses. In cases where the metaphase plate moved/shifted in total two separate measurements were performed and the mean was taken for the analysis. The distance versus time plots showing the displacement of a KT from the metaphase plate were created as previously described [4] . For the change in dynamic localization of GFP-Kif18A ( Fig. 6e ), pixel intensities of Kif18A at the KT area or along the microtubule lattice were quantified as described for the analysis of Kif18A localization in fixed cells. The mean was calculated for the indicated time points. All data were analysed in Microsoft Excel and Origin (Originlab). To determine statistical significance a two-tailed, unpaired Student’s t -test using Excel was performed. Inhibitor and phosphatase treatment Cells (5 × 10 6 ) were seeded in thymidine for 20 h and released by washout. After 2 h, nocodazole was added for 16 h. Cells were collected by mitotic shake-off, released by PBS wash. After drug treatment cells were collected, washed with PBS and lysed (25 mM Tris pH 7.4, 300 mM NaCl, 5 mM EDTA, 0.5% Triton-X-100, 10 U ml −1 DNase1 (Sigma), 20 mM β-Glycerophosphate, 20 mM NaF, 0.3 mM NaV, 1 mM DTT and complete EDTA-free protease inhibitors (Roche)) for 30 min on ice. Cell lysate was cleared by centrifugation at 4 °C for 30 min at 20,000 g and SDS sample buffer was added. Small molecule inhibitors were used as follows: 2 mM or 5 mM thymidine (Sigma), 500 nM nocodazole (Sigma), 20 μM MG132 (Cayman), 100 μM roscovitine (Sigma), 10 or 50 μM RO-3306 (Santa Cruz) and 20 μM VS-83 (ref. 32 ). For the phosphatase treatment 1 U μl −1 CIP was added to cell extracts in CIP-buffer (25 mM Tris pH 8.0, 300 mM NaCl, 0.5% Triton-X-100, 1 mM MgCl 2 , 10 U ml −1 DNase1 (Sigma), 1 mM DTT and protease inhibitors (Roche)) and incubated for 1 h at 37 °C. The reaction was stopped by addition of SDS sample buffer. For cell extracts in Supplementary Fig. 1b , cells were collected and resuspended in SDS sample buffer. For lambda phosphatase treatment, cells were lysed (25 mM Tris pH 7.4, 300 mM NaCl, 0.5% Triton-X-100, 10 U ml −1 DNase1 (Sigma), 1 mM MnCl 2 , 1 mM DTT and complete EDTA-free protease inhibitors (Roche)). The cleared supernatant was incubated for 30 min with 12.5 ng μl −1 lambda phosphatase at 30 °C. Immunoblotting For western blot analyses, antibodies were used as follows: affinity-purified anti-human Kif18A antibodies [24] , affinity-purified anti phospho-specific pS674 and pS684 Kif18A (peptide sequences see below; 1:300; rabbit); anti-human cyclin B1 (1:3,000; Millipore, 05-373); anti-human cyclin A (1:200; Santa Cruz, sc-751), anti-tubulin DM1α (1:1000; Sigma, T6199); affinity-purified anti-human Cdc27 (1:500; C-terminal peptide); anti-GFP (1:1,000; Covance, MMS-118P); anti-human PP1α (1:500; Millipore, 07-273); anti-human PP1γ1 (1:500; Millipore, 07-1218). Horseradish-peroxidase-conjugated anti-rabbit or anti-mouse (1:3000; Dianova) were used as secondary antibodies. Full uncropped scans of all western blots are provided in Supplementary Figs 3–5 . GFP immunoprecipitation HeLa cells (5 × 10 6 ) were seeded and 24 h later transfected with GFP, GFP-PP1α or GFP-PP1γ. Twenty-four hours after transfection, cells were synchronized as described above and blocked in mitosis for 1 h by treatment with 20 μM MG132. Cells were lysed (25 mM Tris pH 7.4, 300 mM NaCl, 5 mM EGTA, 0.5% Triton-X-100, 1 mM MnCl 2 , 1 mM MgCl 2 , 20 U ml −1 DNase1 (Sigma), 20 mM β-Glycerophosphate, 20 mM NaF, 0.3 mM NaV, 1 mM DTT and complete EDTA-free protease inhibitors (Roche)) and incubated for 30 min at 4 °C. After 20,000 g centrifugation for 30 min, the cleared supernatant was recovered. Lambda phosphatase treatment was performed as described above. 250μg GFP-binding protein was coupled to sulfo-link beads (Pierce) according to the manufacturer’s protocol and incubated with the cleared supernatant for 3 h at 4 °C. The beads were washed three times with lysis buffer and bound proteins were eluted with SDS sample buffer. Phosphopeptide antibody production and affinity purification Two synthetic phosphopeptides (C-RRKLMPS(p)PLK-amid and TLKS(p)PPSQSV-C-amid) of human Kif18A were generated by Peptide-Speciality-Laboratories GmbH (Heidelberg). Phospho-specific pS674 and pS684 Kif18A antibodies were generated in rabbits and affinity-purified using the phosphopeptide coupled to Sulfo-link coupling resin (Pierce). Protein purification GST-tagged Kif18A fragments were expressed in BL21(DE3)-RIL cells and purified according standard protocols (GE Healthcare). For purification of PP1, catalytic isoforms alpha (NM_002710, transcript variant 1) and gamma (NM_002710, transcript variant 1) were expressed as His-tagged constructs in BL21(DE3)-RIL. Bacteria were grown at 37 °C to optical density 0.5 before induction with 0.5 mM isopropyl-β- D -thiogalactoside for 4 h at 37 °C in the presence of 1 mM MnCl 2 . Cells were collected and purified using Ni-IDA (Macherey and Nagel) in accordance with the manufacturer’s protocol, except that instead of phosphate buffer a Hepes-buffer (50 mM Hepes pH 8.0, 300 mM NaCl, 1 mM MnCl 2 ) was used. In the lysis- and wash- buffer, 0.1% TX-100 and complete EDTA-free protease inhibitors (Roche) were included. Eluted fractions were dialysed overnight in 50 mM Hepes pH 7.5, 200 mM NaCl, 1 mM MnCl 2 , 2.5 mM DTT, 0.1 mM EGTA, 20% glycerol and 0.025% Tween-20. His-GFP-Kif18A variants were purified as described previously [24] , except for the lambda phosphatase treatment: 100 ng ml −1 lambda phosphatase was added in wash-buffer supplemented with 2 mM MnCl 2 to the beads after binding and the first washing step. The beads were incubated for 30 min at RT. Kinase assay with cell extract Kinase assays were performed as described in Fig. 1i . HeLa cells (1.5 × 10 7 ) were seeded in 2 mM thymidine for 20 h. Cells were released from thymidine and 2 h after the release, nocodazole or RO-3306 was added for 16 h. RO-3306 treated cells were released by washing with pre-warmed PBS and incubated for additional 20 min. Cells were collected mitotic shake-off, washed with PBS and lysed (50 mM Tris pH 7.4, 150 mM NaCl, 5 mM EGTA, 1.0% NP-40, 1 mM MgCl 2 , 10 U ml −1 DNase 1 (Thermo Scientific), 40 mM β-Glycerophosphate, 40 mM NaF, 0.6 mM NaV, 1 mM DTT and complete EDTA-free protease inhibitors (Roche)) and incubated for 30 min at 4 °C. GST-Kif18A CT,WT (0.5 μg) were coupled to Glutathione-Magnetic-Beads (Thermo Scientific) for 60 min in TBS-T at RT. After washing with lysis buffer, the beads were equally distributed and incubated with cleared supernatant of the cell lysate supplemented with 10 μM MgATP and where indicated with 50 μM RO-3306. The reactions were incubated at 25 °C. GST-Kif18A CT bound complexes were washed and eluted from the beads with SDS sample buffer. In vitro pull-down experiments 5μg of GST-Kif18A CT (WT or mutants) were coupled to Glutathione-Magnetic-Beads (Thermo Scientific) for 60 min in TBS-T at RT. After washing (50 mM Tris pH 7.5, 150 mM NaCl, 1 mM DTT, 1 mM MgCl 2 , 1 mM MnCl 2 , 0.1 mM MgATP, 0.1% TX-100, 10% Glyerol), beads were equally distributed and 5 μg bacterially purified His-PP1α or -PP1γ were added in binding buffer and incubated for 2 h at 4 °C. GST-Kif18A CT bound complexes were washed with binding buffer and eluted from the beads with SDS sample buffer. In vitro kinase assay In vitro kinase assays were performed at 30 °C (10 mM Tris pH 7.5, 10 mM MgCl 2 and 1 mM DTT) for 30 min. Phosphorylation of WT GST-Kif18A NT/CT ( Fig. 1e ) were performed by incubation of 25 ng μl −1 protein with 3 ng μl −1 Cdk1/cyclin B1 in the presence of 0.1 mM MgATP and 0.4 μCi/μl γ- 32 P ATP. GST-Kif18A CT mutants (40 ng μl −1 ) ( Fig. 1g ) were phosphorylated with 1.8 ng μl −1 Cdk1/cyclin B1, 0.1 mM MgATP and 0.2 μCi/μl γ- 32 P ATP. Kinase reactions were stopped with SDS sample buffer. For Supplementary Fig. 1g , the kinase assay was performed in Hepes-buffer (25 mM Hepes pH 7.5, 10 mM MgCl 2 , 5 mM EGTA and 1 mM DTT) with 25 ng μl −1 GST-Kif18A CT WT or mutant proteins, 1.8 ng μl −1 Cdk1/cyclin B1 and 1 mM MgATP. In vitro phosphatase assay GST-Kfi18A CT WT or PP1-binding mutant were prephosphorylated with Cdk1/cyclin B1 (30 min at 30 °C in Tris-buffer, 6 ng μl −1 GST-Kif18A, 0.2 mM MgATP and 3 ng μl −1 Cdk1/cyclin B1). For the in vitro phosphatase assay, PP1α or PP1γ in phosphatase-buffer (25 mM Tris pH 7.5, 150 mM NaCl, 1 mM DTT, 1 mM MnCl 2 ) were added into the kinase reaction (without removing Cdk1/cyclin B1) resulting in final concentrations of 16 mM Tris pH 7.5, 60 mM NaCl, 1 mM MnCl 2 , 6 mM MgCl 2 , 1 mM DTT and 0.1 mM MgATP. The reaction was incubated at 30 °C for additional 15 min or 30 min, stopped with SDS sample buffer. Mass spectrometry In vitro kinase assays of GST-Kif18A CT were performed with active or heat-inactivated Cdk1/cyclin B1. The sample with inactive kinase served as background control. After In-gel Pepsin-digestion, the extracted peptides were analysed by reversed phase liquid chromatography nanospray tandem mass spectrometry using an LTQ-Orbitrap mass spectrometer (Thermo Fisher) and an Eksigent nano-HPLC. Tandem mass spectra were searched against the Swissprot human protein database using Mascot (Matrix Science) using static cysteine alkylation by iodoacetamide and variable methionine oxidation. In vitro gliding assay GMPCPP-stabilized MTs were polymerized in BRB80 and 1 mM GMPCPP as described previously [24] , except that the polymerized MTs were resuspended in BRB80 supplemented with 10 μM taxol. Purified His-GFP-Kif18A WT was incubated with 10 ng μl −1 Cdk1/cyclin B1 (20 mM Tris pH 7.4 and 1 mM MgATP) for 20 min at 30 °C. One half of the kinase reaction was stopped by addition of SDS sample buffer. The other half of the reaction was floated in the motility chamber. For motility assays, prephosphorylated protein was immobilized to cover slips as described [24] . Movement of attached MTs was observed with a Plan 100 × 1.4 DIC Plan Apochromat oil objective (Zeiss) on a Axio Imager.M1 (Zeiss) equipped with a HXP 120 and a Cascade II:512 EMCCD camera (Photometrics). Images were analysed using ImageJ and the velocity (μm min −1 ) was calculated from kymographs generated on moving MTs. How to cite this article: Häfner, J. et al . Pre-anaphase chromosome oscillations are regulated by the antagonistic activities of Cdk1 and PP1 on Kif18A. Nat. Commun. 5:4397 doi: 10.1038/ncomms5397 (2014).